RECQ5-dependent SUMOylation of DNA topoisomerase I prevents transcription-associated genome instability DNA topoisomerase I (TOP1) has an important role in maintaining DNA topology by relaxing supercoiled DNA. Here we show that the K391 and K436 residues of TOP1 are SUMOylated by the PIAS1–SRSF1 E3 ligase complex in the chromatin fraction containing active RNA polymerase II (RNAPIIo). This modification is necessary for the binding of TOP1 to RNAPIIo and for the recruitment of RNA splicing factors to the actively transcribed chromatin, thereby reducing the formation of R-loops that lead to genome instability. RECQ5 helicase promotes TOP1 SUMOylation by facilitating the interaction between PIAS1, SRSF1 and TOP1. Unexpectedly, the topoisomerase activity is compromised by K391/K436 SUMOylation, and this provides the first in vivo evidence that TOP1 activity is negatively regulated at transcriptionally active chromatin to prevent TOP1-induced DNA damage. Therefore, our data provide mechanistic insight into how TOP1 SUMOylation contributes to genome maintenance during transcription. The prevention and efficient repair of DNA double-stranded breaks (DSBs) is important for genome integrity in order to prevent cell death or cellular transformation, which is a precursor for cancer development. DSBs can form as a result of exposure to DNA-damaging agents, but they can also arise during normal cellular processes. For example, emerging models suggest that unusual nucleic acid structures, such as extensive RNA:DNA hybrids, known as R-loops, which form during transcription between the newly synthesized RNA and the DNA template strand, are naturally occurring roadblocks for DNA replication forks, leading to fork collapse and DSB formation [1] , [2] . Nonetheless, even though R-loop formation can lead to genome instability, the R-loop is a key structure for programmed genome rearrangements, transcription termination and the maintenance of unmethylated CpG islands [3] , [4] , [5] . Therefore, the R-loop has both positive and negative consequences to DNA metabolism and should be tightly regulated. R-loop formation may be facilitated by highly G-C-rich sequences and the negative supercoiling of DNA that occurs during transcription [6] , [7] . One proposed way the cell could prevent R-loop formation is for DNA topoisomerase I (TOP1) to relax the transcriptionally generated supercoiled DNA [2] . However, there is the corresponding risk of TOP1-induced DSBs and mutations at highly transcribed loci due to the accumulation of trapped TOP1–DNA covalent complexes caused by naturally aborted topoisomerase reactions or by the treatment with TOP1 poisons [8] . Alternatively, mRNA processing and transport may assist in preventing R-loops [9] , because the binding of splicing factors to the nascent RNA transcript may prevent the RNA from invading the DNA template [2] . Furthermore, by excising introns from the pre-mRNA, the homology between the newly synthesized mRNA and the DNA template is reduced, and this could decrease the stability of RNA:DNA hybrid. Consistent with this model, a defect in the splicing factor SRSF1 (also known as ASF/SF2) causes R-loop-induced DSBs [10] , but overexpressing the RNPS1 RNA binding protein reverses the DSB accumulation seen in SRSF1-depleted cells [11] . Interestingly, a recent study demonstrated that TOP1 is required for SRSF1-dependent R-loop avoidance [1] . However, the mechanism that collaborates TOP1 with RNA processing factors to prevent R-loops has remained unknown. Human RECQ5, a member of the highly conserved RECQ family of DNA helicases and a tumour suppressor [12] , is a stable RNA polymerase II (RNAPII)-interacting protein in vivo [13] , [14] . RECQ5 is important for preventing both transcription-associated DSBs and DSBs induced by TOP1 poisons, such as camptothecin (CPT) [15] , [16] , [17] . The increased DSB formation observed in Recq5- deficient cells may contribute to elevated frequencies of homologous recombination and genome rearrangements [12] , [16] . RECQ5 prevents transcription-associated DSBs by suppressing RNAPII-dependent transcription initiation [18] , and this may be achieved by the interaction between RNAPII and the RECQ5 KIX domain, which blocks the binding of transcription elongation factor TFIIS to RNAPII [19] . RECQ5 is also known to interact with the active RNAPII (RNAPIIo) elongation complex to maintain the transcription elongation rate and prevent genome instability [15] , [20] , [21] . However, the exact mechanism by which RECQ5 maintains genome stability during transcription elongation has also not been determined. Here we report a novel function of RECQ5 in suppressing R-loop-mediated genome instability. We have discovered that the helicase domain of RECQ5 interacts directly with TOP1 and facilitates TOP1 SUMOylation at lysine (K) 391 and 436 residues at highly transcribed loci in a manner that is dependent on the PIAS1 E3 ligase and its cofactor SRSF1. K391/K436 SUMOylation promotes the interaction of TOP1 with RNAPIIo and is necessary for the efficient recruitment of mRNA processing factors to the transcriptionally active chromatin to prevent R-loops. This function explains why RECQ5-mutant cells defective in K391/K436 SUMOylation accumulate R-loops and R-loop-induced DSBs. In addition, we further demonstrate that K391/K436 SUMOylation significantly reduces the catalytic activity of TOP1, indicating that TOP1-dependent relaxation of negatively supercoiled DNA is unlikely to contribute to R-loop prevention at highly transcribed gene loci. This negative regulation of TOP1 activity may be necessary to prevent the accumulation of trapped TOP1–DNA complexes at these regions and genome instability [12] , [17] . TOP1 is SUMOylated at K391 and K436 during transcription To enrich for TOP1 molecules associated with actively transcribed gene loci for our analysis, we modified our standard chromatin fractionation protocol [15] . Briefly, after removing cytoplasmic (Cyt) and non-DNA-bound nuclear proteins from HEK293T cell extracts, the chromatin-bound (CB) pellet was first treated with RNase A, and the solubilized proteins were collected as the CB:RNA+ fraction ( Fig. 1a ). Because RNase A treatment destabilizes open chromatin structures that contain RNAPII-dependent RNAs and active transcription factories [22] , the majority of the RNAPIIo elongation complexes, but not the inactive RNAPIIa, were found in the CB:RNA+ fraction ( Fig. 1b , centre lane; Fig. 1c , top panel; Supplementary Fig. 1 ). The remaining insoluble pellet was further digested with benzonase, and the protein fraction collected after benzonase treatment was designated as CB:RNA− ( Fig. 1a ). In addition to active transcription factories, chromatin remodelling enzymes and DNA replication factors, such as proliferating cell nuclear antigen (PCNA), were also enriched in the CB:RNA+ fraction ( Fig. 1c , fourth panel from top; Supplementary Fig. 1 ). However, when normalized to histone H4 concentrations, only the presence of RNAPIIo and splicing factor U2AF65, but not PCNA, was significantly reduced in the CB:RNA+ fraction after treatment with the RNAPII elongation-specific inhibitor 5,6-dichloro-1-β-D-ribofuranosylbenzimidazole (DRB; Fig. 1c and Supplementary Fig. 1 ). Western blot analysis showed that the CB:RNA− fraction also contained a minor portion of RNAPIIo, relative to the CB:RNA+ fraction, along with the inactive RNAPIIa ( Fig. 1b , right lane; Fig. 1c , right panels; Supplementary Fig. 1 ). These RNAPIIo molecules in the CB:RNA− fraction were likely associated with more compact chromosomal regions that had lower transcription activity and could be converted to RNAPIIa by DRB treatment ( Fig. 1c and Supplementary Fig. 1 ). 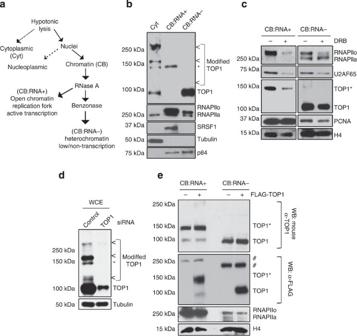Figure 1: Transcription-dependent post-translational modification of TOP1. (a) Schematic diagram of the cell fractionation to separate proteins associated with transcriptionally active open chromatin structure (for example, CB:RNA+) from proteins that are bound to heterochromatin, or from regions not highly transcribed (CB:RNA−). (b) Representative western blot (WB) analysis of RNAPII, splicing factor SRSF1 and TOP1 in cytoplasmic (Cyt), CB:RNA+ and CB:RNA− fractions prepared from 293 T cells. A mouse α-TOP1 antibody was used to detect TOP1. Tubulin and p84 were used as fractionation controls. Protein bands marked with ‘<’ or ‘*’ are potential modified forms of TOP1. (c) Representative WB analysis of RNAPII, splicing factor U2AF65, TOP1 and replication factor PCNA in CB:RNA+ and CB:RNA- fractions prepared from 293 T cells with or without treatment with the transcription inhibitor DRB (25 μM, 1 h). Histone H4 was used as the loading control, and a mouse α-TOP1 antibody was used to detect TOP1. (d) Representative WB analysis of TOP1 in whole-cell extracts (WCEs) prepared from control or TOP1 siRNA-treated cells. A mouse α-TOP1 antibody was used to detect TOP1. (e) Representative WB analysis using a mouse α-TOP1 antibody (upper panel) and mouse α-FLAG antibody (centre panel) to detect endogenous TOP1 and exogenously expressed FLAG-TOP1 in CB:RNA+ and CB:RNA− fractions prepared from 293 T cells transfected with pCMV vector alone or the pCMV-FLAG-TOP1 plasmid. Protein bands marked with ‘#’ are nonspecific crossreactivity by the mouse α-FLAG antibody. RNAPII and Histone H4 were used as the loading controls. Figure 1: Transcription-dependent post-translational modification of TOP1. ( a ) Schematic diagram of the cell fractionation to separate proteins associated with transcriptionally active open chromatin structure (for example, CB:RNA+) from proteins that are bound to heterochromatin, or from regions not highly transcribed (CB:RNA−). ( b ) Representative western blot (WB) analysis of RNAPII, splicing factor SRSF1 and TOP1 in cytoplasmic (Cyt), CB:RNA+ and CB:RNA− fractions prepared from 293 T cells. A mouse α-TOP1 antibody was used to detect TOP1. Tubulin and p84 were used as fractionation controls. Protein bands marked with ‘<’ or ‘*’ are potential modified forms of TOP1. ( c ) Representative WB analysis of RNAPII, splicing factor U2AF65, TOP1 and replication factor PCNA in CB:RNA+ and CB:RNA- fractions prepared from 293 T cells with or without treatment with the transcription inhibitor DRB (25 μM, 1 h). Histone H4 was used as the loading control, and a mouse α-TOP1 antibody was used to detect TOP1. ( d ) Representative WB analysis of TOP1 in whole-cell extracts (WCEs) prepared from control or TOP1 siRNA-treated cells. A mouse α-TOP1 antibody was used to detect TOP1. ( e ) Representative WB analysis using a mouse α-TOP1 antibody (upper panel) and mouse α-FLAG antibody (centre panel) to detect endogenous TOP1 and exogenously expressed FLAG-TOP1 in CB:RNA+ and CB:RNA− fractions prepared from 293 T cells transfected with pCMV vector alone or the pCMV-FLAG-TOP1 plasmid. Protein bands marked with ‘#’ are nonspecific crossreactivity by the mouse α-FLAG antibody. RNAPII and Histone H4 were used as the loading controls. Full size image Using this chromatin fractionation protocol, we found that the majority of the 98-kDa TOP1 molecules were present in the CB:RNA− fraction ( Fig. 1b , top panel, third lane; Supplementary Fig. 1 ). However, in the CB:RNA+ fraction, a distinct 145-kDa species (*) recognized by a mouse monoclonal α-TOP1 antibody was observed ( Fig. 1b , top panel, centre lane; Supplementary Fig. 1 ). The presence of TOP1* was reduced in the CB:RNA+ fraction prepared from DRB-treated cells ( Fig. 1c and Supplementary Fig. 1 ) and was eliminated in whole-cell extracts treated with TOP1-specific small interfering RNA (siRNA; Fig. 1d and Supplementary Fig. 1 ). These observations indicated that the 145-kDa TOP1* species is a post-translationally modified form of TOP1, and that its presence in the CB:RNA+ fraction is dependent on RNAPII-mediated transcription. Indeed, exogenously expressed FLAG-TOP1 in the CB:RNA+ fraction also exhibited a similar mobility shift as the endogenous TOP1* on SDS–PAGE ( Fig. 1e and Supplementary Fig. 1 ). Next, we immunopurified the FLAG-TOP1* molecules from the CB:RNA+ fraction ( Fig. 1e and Supplementary Fig. 1 ) and found that the purified FLAG-TOP1* was recognized by an α-SUMO1 antibody ( Fig. 2a and Supplementary Fig. 2 ). Treatment with SUMO-deconjugating enzyme, SENP1, efficiently converted TOP1* to the unmodified form of TOP1 ( Fig. 2a , compare centre and right lanes; Supplementary Fig. 2 ), confirming that the TOP1* molecule is SUMOylated (SUMO-TOP1). 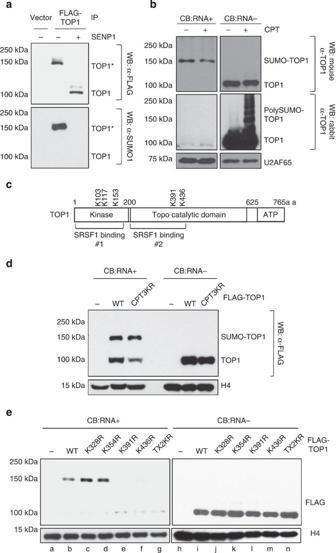Figure 2: Transcription-dependent TOP1 K391/K436 SUMOylation. (a) FLAG-TOP1 was immunopurified with M2 agarose from the CB:RNA+ fractions of the 293 T cells, treated with or without SENP1, and analysed on WBs probed with mouse α-FLAG (top) and mouse α-SUMO1 (bottom). (b) Representative WB analysis of TOP1 using a mouse α-TOP1 antibody (top) and a rabbit α-TOP1 antibody (centre) in the CB:RNA+ and CB:RNA− fractions prepared from 293 T cells with or without CPT treatment (5 μM for 30 min, followed by 4 h recovery in medium without CPT). Splicing factor U2AF65 was used as the loading control. (c) Diagram of human TOP1, its known catalytic domains (kinase, topoisomerase and ATP binding) and SRSF1-interacting domains. CPT-dependent SUMOylation sites (K103, K117 and K153) and transcription-induced SUMOylation sites (K391 and K436) are shown. (d) WB analysis of FLAG-TOP1 WT and the CPT3KR mutant containing the K103R, K117R and K153R mutations in the CB:RNA+ and CB:RNA− fractions. Histone H4 was used as the loading control. (e) WB analysis of FLAG-TOP1 WT and the K328R, K354R, K391R, K436R and TX2KR (K391R+K436R) mutants in the CB:RNA+ and CB:RNA−- fractions. Histone H4 was used as the loading control. The K328, K354, K391 and K436 residues are located within the topoisomerase domain of TOP1. Figure 2: Transcription-dependent TOP1 K391/K436 SUMOylation. ( a ) FLAG-TOP1 was immunopurified with M2 agarose from the CB:RNA+ fractions of the 293 T cells, treated with or without SENP1, and analysed on WBs probed with mouse α-FLAG (top) and mouse α-SUMO1 (bottom). ( b ) Representative WB analysis of TOP1 using a mouse α-TOP1 antibody (top) and a rabbit α-TOP1 antibody (centre) in the CB:RNA+ and CB:RNA− fractions prepared from 293 T cells with or without CPT treatment (5 μM for 30 min, followed by 4 h recovery in medium without CPT). Splicing factor U2AF65 was used as the loading control. ( c ) Diagram of human TOP1, its known catalytic domains (kinase, topoisomerase and ATP binding) and SRSF1-interacting domains. CPT-dependent SUMOylation sites (K103, K117 and K153) and transcription-induced SUMOylation sites (K391 and K436) are shown. ( d ) WB analysis of FLAG-TOP1 WT and the CPT3KR mutant containing the K103R, K117R and K153R mutations in the CB:RNA+ and CB:RNA− fractions. Histone H4 was used as the loading control. ( e ) WB analysis of FLAG-TOP1 WT and the K328R, K354R, K391R, K436R and TX2KR (K391R+K436R) mutants in the CB:RNA+ and CB:RNA−- fractions. Histone H4 was used as the loading control. The K328, K354, K391 and K436 residues are located within the topoisomerase domain of TOP1. Full size image The ∼ 50-kDa increase in the molecular weight of SUMO-TOP1 compared with non-modified TOP1 suggested that SUMO-TOP1 contained 2–3 SUMO conjugates and our next goal was to identify the key amino acids for this modification. SUMOplot analysis predicted that human TOP1 contains 12 motifs that have high probabilities for SUMOylation, and TOP1 has been shown to be poly-SUMOylated at K103, K117 and K153 in response to CPT [23] , [24] , [25] , [26] . However, we found that transcription-associated TOP1 SUMOylation is distinct from the SUMOylation events induced by CPT. First, the level of SUMO-TOP1 in the CB:RNA+ fraction did not increase after CPT treatment ( Fig. 2b , top left panel; Supplementary Fig. 2 ). Second, the CPT-induced modifications and the transcription-induced SUMOylation were recognized by different α-TOP1 antibodies, suggesting that these modifications affect different epitopes of the TOP1 protein. For example, the mouse monoclonal α-TOP1 antibody that recognized the SUMO-TOP1 in the CB:RNA+ fraction failed to react with CPT-induced modified forms of TOP1 ( Fig. 2b , top right panel; Supplementary Fig. 2 ), which was only detected in the CB:RNA− fraction using a rabbit α-TOP1 antibody ( Fig. 2b , right panels; Supplementary Fig. 2 ). Conversely, the rabbit α-TOP1 antibody did not recognize the TOP1 that was modified by the transcription-induced SUMOylation ( Fig. 2b , left panels; Supplementary Fig. 2 ). Finally, we transiently expressed a FLAG-TOP1-CPT3KR construct containing K103R, K117R and K153R mutations in HEK293T cells to test whether these mutations abolished transcription-associated SUMOylation of TOP1 ( Fig. 2c ). Unlike the endogenous TOP1, which only exists as the SUMOylated form in the CB:RNA+ fraction, the non-modified form of FLAG-TOP1, when transiently expressed at higher levels, could sometimes be found in the CB:RNA+ fraction along with the SUMOylated FLAG-TOP1 ( Fig. 2d and Supplementary Fig. 3 ). Nonetheless, we found that these mutations in the CPT3KR mutant did not abolish TOP1 SUMOylation in the CB:RNA+ fraction ( Fig. 2d and Supplementary Fig. 3 ). Instead, mutation analyses revealed that K391R and K436R single mutations and a K391R/K436R double mutation (TX2KR) abolished TOP1 SUMOylation in the CB:RNA+ fraction without affecting the non-modified form of TOP1 in the CB:RNA− fraction ( Fig. 2e , lanes e–g and l–n; Supplementary Figs 3 and 4 ). These data together demonstrate that K391 and K436 residues are important for the SUMOylation of the TOP1 molecules associated with highly transcribed regions of chromatin. RECQ5-SRSF1-PIAS1-dependent TOP1 K391/K436 SUMOylation We next wanted to discover the enzymes responsible for K391 and K436 TOP1 SUMOylation. Several enzymes have been implicated in SUMOylating TOP1. For example, the E3 ligase TOPORS adds poly-SUMO1 groups to TOP1 in response to CPT [23] . The RNA splicing factor SRSF1, which acts as a PIAS1 E3 ligase cofactor in cells, also enhances TOP1 SUMOylation in vitro [27] . However, the in vivo relationship between SRSF1 and PIAS1 in TOP1 SUMOylation has been unknown. Because SRSF1 was previously shown to promote in vitro SUMOylation within the first 200 amino acids of TOP1 [27] , we initially predicted that SRSF1 was unlikely responsible for the SUMOylation of K391 and K436, which located downstream of the first 200 amino acids ( Fig. 2c ). Indeed, in vitro, when suboptimal SUMO E1 and E2 ligases were incubated with purified 125 kDa GST-TOP1 fusion proteins, we found that the addition of purified recombinant SRSF1, PIAS1 or both produced a 150-kDa SUMOylated GST-TOP1 species, labelled as SUMO-[GST-TOP1]-150 ( Fig. 3a , lanes b–d and f; Supplementary Fig. 5 ), which was different from the predicted 175 kDa for the K391/K436 SUMOylated GST-TOP1. Furthermore, K391R and K436R double mutations in the GST-TX2KR mutant protein failed to prevent the formation of SUMO-[GST-TOP1]-150 ( Fig. 3b and Supplementary Fig. 5 ). However, to our surprise, in either SRSF1- or PIAS1-depleted cells, TOP1 K391/K436 SUMOylation was abolished ( Fig. 3c,d , lanes b and c; Supplementary Fig. 6 ), arguing that in vivo SRSF1 and PIAS1 are indeed required but not sufficient for this reaction. 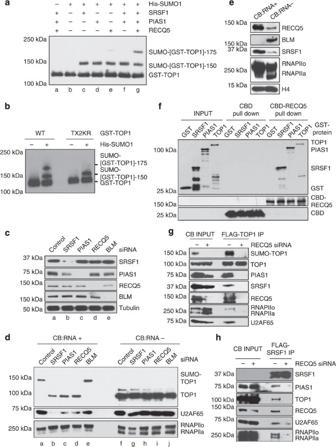Figure 3: RECQ5-SRSF1-PIAS1 induced TOP1 K391/K436 SUMOylation. (a) WB analysis of the recombinant GST-TOP1 after representativein vitroSUMOylation assays in the presence of recombinant His-SUMO1, GST-SRSF1, GST-PIAS1 and CBD-RECQ5. Anti-StrepII antibody, instead of anti-GST antibody, was used to detect GST-TOP1, which was also tagged with StrepII at the C terminus. (b) WB analysis using anti-StrepII antibody to detect the recombinant GST-TOP1 WT and TX2KR mutant after representativein vitroSUMOylation assays in the presence or absence of His-SUMO1. (c) The protein levels of SRSF1, PIAS1, RECQ5 and BLM were analysed in WCEs prepared from control, SRSF1, PIAS1, RECQ5 and BLM siRNA knockdown cells. Tubulin was used as the loading control. (d) WB analysis of RNAPII, splicing factor U2AF65 and TOP1 in CB:RNA+ and CB:RNA− fractions prepared from the cells inc. (e) Representative WB analysis of the distribution of RECQ5 and BLM in CB:RNA+ and CB:RNA− fractions. SRSF1 and RNAPII are shown as fractionation controls. Histone H4 was used as loading control. (f) Representative WB analysis for the presence of the recombinant GST, GST-SRSF1, GST-PIAS1 and GST-TOP1 before (INPUT) and afterin vitropull-down reactions using CBD (centre four lanes) or CBD-RECQ5 (right 4 lanes) conjugated to chitin beads. (g) Representative WB analysis of SUMO-FLAG-TOP1, FLAG-TOP1, PIAS1, SRSF1, RECQ5, RNAPII and U2AF65 in the CB fraction (two left lanes) and immunopurified FLAG-TOP1 complexes (two right lanes) from the CB fractions prepared from 293 T cells with or without RECQ5 siRNA-based depletion. FLAG-TOP1 proteins were detected using rabbit α-FLAG antibody. (h) Representative WB analysis of TOP1, PIAS1, FLAG-SRSF1, RECQ5, RNAPII and U2AF65 in the CB INPUT (2 left lanes) and immunopurified FLAG-SRSF1 complexes (2 right lanes) from the CB fractions prepared from 293 T cells with or without RECQ5 depletion. FLAG-SRSF1 proteins were detected using rabbit α-FLAG antibody. Figure 3: RECQ5-SRSF1-PIAS1 induced TOP1 K391/K436 SUMOylation. ( a ) WB analysis of the recombinant GST-TOP1 after representative in vitro SUMOylation assays in the presence of recombinant His-SUMO1, GST-SRSF1, GST-PIAS1 and CBD-RECQ5. Anti-StrepII antibody, instead of anti-GST antibody, was used to detect GST-TOP1, which was also tagged with StrepII at the C terminus. ( b ) WB analysis using anti-StrepII antibody to detect the recombinant GST-TOP1 WT and TX2KR mutant after representative in vitro SUMOylation assays in the presence or absence of His-SUMO1. ( c ) The protein levels of SRSF1, PIAS1, RECQ5 and BLM were analysed in WCEs prepared from control, SRSF1, PIAS1, RECQ5 and BLM siRNA knockdown cells. Tubulin was used as the loading control. ( d ) WB analysis of RNAPII, splicing factor U2AF65 and TOP1 in CB:RNA+ and CB:RNA− fractions prepared from the cells in c . ( e ) Representative WB analysis of the distribution of RECQ5 and BLM in CB:RNA+ and CB:RNA− fractions. SRSF1 and RNAPII are shown as fractionation controls. Histone H4 was used as loading control. ( f ) Representative WB analysis for the presence of the recombinant GST, GST-SRSF1, GST-PIAS1 and GST-TOP1 before (INPUT) and after in vitro pull-down reactions using CBD (centre four lanes) or CBD-RECQ5 (right 4 lanes) conjugated to chitin beads. ( g ) Representative WB analysis of SUMO-FLAG-TOP1, FLAG-TOP1, PIAS1, SRSF1, RECQ5, RNAPII and U2AF65 in the CB fraction (two left lanes) and immunopurified FLAG-TOP1 complexes (two right lanes) from the CB fractions prepared from 293 T cells with or without RECQ5 siRNA-based depletion. FLAG-TOP1 proteins were detected using rabbit α-FLAG antibody. ( h ) Representative WB analysis of TOP1, PIAS1, FLAG-SRSF1, RECQ5, RNAPII and U2AF65 in the CB INPUT (2 left lanes) and immunopurified FLAG-SRSF1 complexes (2 right lanes) from the CB fractions prepared from 293 T cells with or without RECQ5 depletion. FLAG-SRSF1 proteins were detected using rabbit α-FLAG antibody. Full size image RECQ5, which was primarily found in the CB:RNA+ fraction ( Fig. 3e and Supplementary Fig. 7 ), is important for providing resistance to both transcription- and TOP1-induced genome instability [13] , [14] , [15] , [17] . Interestingly, we found that similar to SRSF1 and PIAS1 knockdown, RECQ5 depletion also abolished TOP1 K391/K436 SUMOylation, and this defect is specific to RECQ5 but not other RECQ family DNA helicases, such as BLM ( Fig. 3c,d , lanes d and e; Supplementary Fig. 6 ), which, unlike RECQ5, was mainly found in the CB:RNA− fraction ( Fig. 3e and Supplementary Fig. 7 ). Because in vitro- purified recombinant RECQ5 can interact directly with SRSF1, PIAS1 and TOP1 ( Fig. 3f and Supplementary Fig. 7 ), we hypothesized that RECQ5 may function as a scaffold protein to promote the interactions among SRSF1, PIAS1 and TOP1. Indeed, in the absence of RECQ5, interactions between TOP1-SRSF1, SRSF1-PIAS1 and PIAS1-TOP1 were compromised ( Fig. 3g,h and Supplementary Figs 8, 9 and 10a,b ). Interestingly, the interaction of RECQ5 with TOP1, but not with RNAPII, depended on the presence of SRSF1 ( Supplementary Fig. 10c,d ) and vice versa ( Supplementary Fig. 10e,f ), suggesting that RECQ5, TOP1, SRSF1 and PIAS1 form a complex together, and formation of this complex requires all the components. When we combined RECQ5, TOP1, SRSF1 and PIAS1 in the in vitro SUMOylation assay, we found that an additional SUMOylated TOP1 species (for example, SUMO-[GST-TOP1]-175) with a molecular weight similar to that for the predicted K391/K436 SUMOylated GST-TOP1 was generated ( Fig. 3a , lane g; Supplementary Fig. 5 ). Importantly, the TX2KR mutations abolished the formation of SUMO-[GST-TOP1]-175 ( Fig. 3b and Supplementary Fig. 5 ), confirming that SUMO-[GST-TOP1]-175 was SUMOylated at K391 and K436. All together, our results identified RECQ5 as a novel factor that interacts with TOP1, SRSF1 and PIAS1 to facilitate TOP1 K391/K436 SUMOylation both in vitro and in vivo . K391/K436 SUMOylation promotes TOP1-RNAPIIo interaction Interestingly, in RECQ5 knockdown cells, TOP1 not only failed to interact with the PIAS1–SRSF1 E3 ligase complex but also showed significantly weakened interaction with the RNAPIIo transcription machinery and RNA processing factors, such as U2AF65 ( Fig. 3g and Supplementary Fig. 8 ), suggesting that K391/K436 SUMOylation was responsible for stable interaction with the RNAPIIo elongation complex. Indeed, even though TX2KR mutant was not SUMOylated ( Fig. 4a , top panel; Supplementary Fig. 11 ), it remained capable of interacting with PIAS1 ( Fig. 4a , bottom panel; Supplementary Fig. 11 ), but not RNAPIIo and U2AF65 on human chromatin ( Fig. 4a , third and fourth panels from the top; Supplementary Fig. 11 ). We further demonstrated the effect of K391/K436 SUMOylation on the TOP1-RNAPIIo interaction using in vitro pull-down experiments. For this, we first SUMOylated GST-TOP1 with His-SUMO1 in the presence of RECQ5, PIAS1 and SRSF1 (similar to Fig. 3a , lane g). We then used nickel-nitrilotriacetic acid (Ni-NTA) resin to pull down the His-SUMO. The SUMOylated GST-TOP1 proteins were then eluted from the Ni-NTA resin, immobilized on glutathione beads and treated without or with SENP1 to remove SUMO modifications. The treated glutathione beads containing either GST, modified GST-TOP1 or unmodified GST-TOP1 were then incubated with RNAPIIo purified from the CB:RNA+ fraction of cells expressing a FLAG-tagged version of the RNAPII subunit RPB3 ( Fig. 4b and Supplementary Fig. 12 ). We found that SUMOylated GST-TOP1, but not GST alone, efficiently pulled down RNAPIIo ( Fig. 4b , compare lanes a and c; Supplementary Fig. 12 ). Importantly, the interaction was abolished when the SUMOylated GST-TOP1 was first treated with SENP1 before the pull down ( Fig. 4b , lane b; Supplementary Fig. 12 ). To further distinguish which of the two SUMOylated GST-TOP1 species is responsible for interacting with RNAPIIo in the pull-down experiment shown in Fig. 4b , we performed a reciprocal pull-down experiment by incubating the products of the in vitro GST-TOP1 SUMOylation reactions ( Fig. 4c , top panel; Supplementary Fig. 12 ) with FLAG antibody-conjugated M2 agarose beads containing either purified FLAG-RNAPII from the CB:RNA+ fraction or FLAG-GFP ( Fig. 4c , bottom panel; Supplementary Fig. 12 ). We found that compared with SUMO-[GST-TOP1]-150, SUMO-[GST-TOP1]-175 was significantly enriched on the M2 agarose beads containing FLAG-RNAPII, but not those containing FLAG-GFP ( Fig. 4c and Supplementary Fig. 12 ). These analyses together demonstrate that K391/K436 SUMOylation promotes the interaction of TOP1 with RNAPIIo elongation complex. 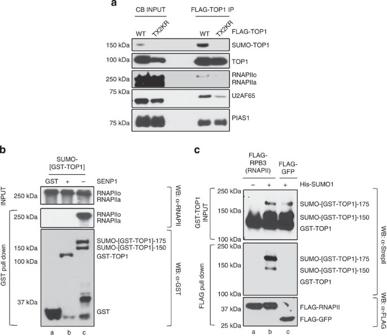Figure 4: K391/K436 SUMOylation promotes TOP1 interactions with RNAPIIo. (a) Representative WB analysis of SUMO-FLAG-TOP1, FLAG-TOP1, PIAS1, RNAPIIo and U2AF65 in the CB INPUT (two left lanes) and the immunopurified FLAG-TOP1 WT or TX2KR complexes (two right lanes) from the CB fractions. FLAG-TOP1 proteins were detected using rabbit α-FLAG antibody. (b) WB analysis for the presence of purified FLAG-RNAPII prepared from CB:RNA+ fraction before (top panel) and after (centre panel) binding to the glutathione beads containing purified GST or SUMOylated GST-TOP1 with or without SENP1 treatment (lower panels). FLAG-RNAPII proteins were detected using rabbit α-RNAPII antibody (top and centre panels), and GST proteins were detected using α-GST antibody (bottom panel). (c) WB analysis using anti-StrepII antibody to detect recombinant GST-TOP1, which was also tagged with StrepII at the C terminus, prepared fromin vitroSUMOylation assays with or without the presence of His-SUMO1 before (top panel) and after (centre panel) binding to the M2 agarose beads containing RNAPII purified using FLAG-RPB3 or FLAG-GFP (lower panel). FLAG-RPB3(RNAPII) and FLAG-GFP proteins were detected using rabbit α-FLAG antibody. Figure 4: K391/K436 SUMOylation promotes TOP1 interactions with RNAPIIo. ( a ) Representative WB analysis of SUMO-FLAG-TOP1, FLAG-TOP1, PIAS1, RNAPIIo and U2AF65 in the CB INPUT (two left lanes) and the immunopurified FLAG-TOP1 WT or TX2KR complexes (two right lanes) from the CB fractions. FLAG-TOP1 proteins were detected using rabbit α-FLAG antibody. ( b ) WB analysis for the presence of purified FLAG-RNAPII prepared from CB:RNA+ fraction before (top panel) and after (centre panel) binding to the glutathione beads containing purified GST or SUMOylated GST-TOP1 with or without SENP1 treatment (lower panels). FLAG-RNAPII proteins were detected using rabbit α-RNAPII antibody (top and centre panels), and GST proteins were detected using α-GST antibody (bottom panel). ( c ) WB analysis using anti-StrepII antibody to detect recombinant GST-TOP1, which was also tagged with StrepII at the C terminus, prepared from in vitro SUMOylation assays with or without the presence of His-SUMO1 before (top panel) and after (centre panel) binding to the M2 agarose beads containing RNAPII purified using FLAG-RPB3 or FLAG-GFP (lower panel). FLAG-RPB3(RNAPII) and FLAG-GFP proteins were detected using rabbit α-FLAG antibody. Full size image K391/K436 SUMOylation reduces TOP1 catalytic activity Human TOP1 is thought to relax supercoiled DNA generated during transcription elongation [2] . Because both K391 and K436 are located within the topoisomerase domain of TOP1 ( Fig. 2c ), we next examined the effect of K391/K436 SUMOylation on the catalytic activity of TOP1. For this, we immunopurified the SUMOylated FLAG-TOP1 wild type (WT) and the SUMOylation-defective TX2KR mutant from the CB:RNA+ fractions using FLAG antibody-conjugated M2 agarose ( Fig. 5a and Supplementary Fig. 13 ). When equal amounts of the purified WT and TX2KR mutant proteins were incubated with the supercoiled DNA substrates, we found that the non-modified TX2KR mutant relaxed the majority of the supercoiled DNA within 10 min of incubation, while it took 40–80 min for the WT proteins to relax the same amount of the DNA ( Fig. 5b ). Consistent with this observation, we carried out topoisomerase reaction using an aliquot of the purified FLAG-TOP1 WT sample that had been first treated with or without SENP1 to remove the SUMO modifications ( Fig. 2a and Supplementary Fig. 2 ), and found that a robust TOP1 catalytic activity was detected when the purified FLAG-TOP1 WT protein sample was pre-treated with SENP1 ( Fig. 5c ). These results indicated that K391/K436 SUMOylation suppresses TOP1 catalytic activity. 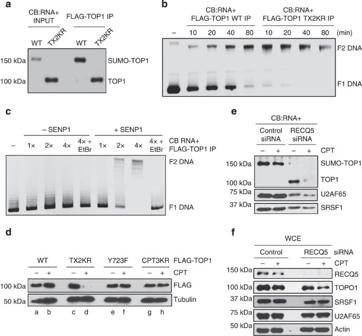Figure 5: K391/K436 SUMOylation inhibits TOP1 catalytic activity. (a) WB analysis of FLAG-TOP1 WT and TX2KR in the CB:RNA+ fractions (two left lanes) and after immunopurification using M2 agarose beads (two right lanes). (b) Equal amounts of purified FLAG-TOP1 WT or TX2KR mutant fromawere assayed for DNA relaxation activity using a supercoiled circular plasmid. The reactions were stopped at the indicated times and analysed on a 1% agarose gel. F1 DNA represented negative supercoiled DNA and F2 DNA represented relaxed circular DNA. (c) Equal amounts of purified FLAG-TOP1 WT with or without SENP1 treatment fromFig. 2awere incubated with supercoiled circular plasmids for 30 min to assay for DNA relaxation activity. The reactions were analysed on a 1% agarose gel. Ethidium bromide was used to inhibit the reaction and as a negative control. (d) The protein levels of FLAG-TOP1 WT, TX2KR, topoisomerase-defective Y723F and CPT-induced SUMOylation-defective mutants in WCE with or without CPT treatment were analysed by WB. Tubulin was used as the loading control. (e) Representative WB analysis of TOP1, U2AF65 and SRSF1 in CB:RNA+ fractions prepared from control and RECQ5 siRNA knockdown cells with or without CPT treatment (5 μM for 30 min, followed by 4 h recovery in medium without CPT). (f) The protein levels of RECQ5, TOP1, SRSF1 and U2AF65 in WCE prepared from either control or RECQ5 knockdown cells with or without CPT treatment were analysed by WB. Actin was used as the loading control. Figure 5: K391/K436 SUMOylation inhibits TOP1 catalytic activity. ( a ) WB analysis of FLAG-TOP1 WT and TX2KR in the CB:RNA+ fractions (two left lanes) and after immunopurification using M2 agarose beads (two right lanes). ( b ) Equal amounts of purified FLAG-TOP1 WT or TX2KR mutant from a were assayed for DNA relaxation activity using a supercoiled circular plasmid. The reactions were stopped at the indicated times and analysed on a 1% agarose gel. F1 DNA represented negative supercoiled DNA and F2 DNA represented relaxed circular DNA. ( c ) Equal amounts of purified FLAG-TOP1 WT with or without SENP1 treatment from Fig. 2a were incubated with supercoiled circular plasmids for 30 min to assay for DNA relaxation activity. The reactions were analysed on a 1% agarose gel. Ethidium bromide was used to inhibit the reaction and as a negative control. ( d ) The protein levels of FLAG-TOP1 WT, TX2KR, topoisomerase-defective Y723F and CPT-induced SUMOylation-defective mutants in WCE with or without CPT treatment were analysed by WB. Tubulin was used as the loading control. ( e ) Representative WB analysis of TOP1, U2AF65 and SRSF1 in CB:RNA+ fractions prepared from control and RECQ5 siRNA knockdown cells with or without CPT treatment (5 μM for 30 min, followed by 4 h recovery in medium without CPT). ( f ) The protein levels of RECQ5, TOP1, SRSF1 and U2AF65 in WCE prepared from either control or RECQ5 knockdown cells with or without CPT treatment were analysed by WB. Actin was used as the loading control. Full size image Because CPT prevents the completion of TOP1 reaction, an increase in the TOP1 activity will accelerate the accumulation of TOP1 covalently attached to DNA in the presence of CPT, leading to rapid TOP1 degradation. Consistent with this, the increased activity by the TX2KR mutation significantly destabilized the TX2KR mutant proteins in cells treated with CPT ( Fig. 5d , compare lanes c and d; Supplementary Fig. 13 ). On the other hand, the CPT3KR mutant showed similar stability as the WT and the catalytically defective Y723F mutant ( Fig. 5d , lanes e–h; Supplementary Fig. 13 ), and this is likely because CPT-induced SUMOylation at K103, K117 and K153 does not alter its topoisomerase activity [25] . Similar to the TX2KR mutant proteins ( Fig. 5d , lane d; Supplementary Fig. 13 ), the unmodified TOP1 found in the CB:RNA+ fraction of the RECQ5 knockdown cells was rapidly degraded in the presence of CPT ( Fig. 5e and Supplementary Fig. 14 ), leading to an overall reduction of the TOP1 protein level in the whole-cell extracts ( Fig. 5f and Supplementary Fig. 14 ), a phenomenon that is consistent with the CPT hypersensitivity in RECQ5-depleted cells [17] . Recruitment of RNA processing factors by TOP1 SUMOylation The reduced TOP1 catalytic activity was unexpected because TOP1 has been implicated in removing supercoiled DNA during transcription to minimize R-loop-induced genome instability [2] . The suppression of TOP1 activity by SUMOylation may be necessary to prevent highly transcribed gene loci from accumulating aborted TOP1–DNA covalent complexes, which are mutagenic and toxic to cells if not removed [8] . Nonetheless, recent studies have unveiled an alternative role of TOP1 in minimizing R-loop formation by promoting the assembly of an mRNA–protein complex [1] , [28] . Consistent with this, we found that in the TOP1 knockdown cells ( Fig. 6a and Supplementary Fig. 15 ), the levels of the RNA processing factors, such as SRSF1 and THOC5, were significantly reduced in the CB:RNA+ fraction ( Fig. 6b , compare lanes a and b; Supplementary Fig. 16 ) but not in the CB:RNA− fraction ( Fig. 6b , compare lanes g and h; Supplementary Fig. 16 ). It is possible that at highly transcribed regions, where there is a significantly increased demand for RNA processing factors, active recruitment and enrichment of these factors by TOP1 is required to allow efficient mRNA processing. This reduction in the levels of RNA processing factors in the CB:RNA+ fraction was rescued by the expression of TOP1 WT, Y723F or the CPT3KR mutant ( Fig. 6b , lanes c,e and f; Supplementary Fig. 16 ). On the other hand, the TX2KR mutant failed to facilitate the recruitment, despite the fact that the mutant protein was detected in the CB:RNA+ fraction ( Fig. 6b , lane d; Supplementary Fig. 16 ). This result argues that the presence of TOP1 alone is not enough to facilitate the recruitment of RNA processing factors, but the K391/K436 SUMOylation is important for this function. Consistent with this, in RECQ5-, SRSF1- or PIAS1-depleted cells, the levels of the RNA processing factors, such as U2AF65, were significantly reduced in the CB:RNA+ fractions ( Figs 3d and 5e ). Because SUMOylation also promotes the interaction of TOP1 with RNA processing factors in addition to RNAPIIo ( Figs 3g and 4a ), it is likely that TOP1 facilitates the recruitment of RNA processing factors via protein–protein interactions. Interestingly, in the CB:RNA− fraction in cells expressing the Y723F mutant, we observed a modified form of TOP1 (TOP1**; Fig. 6b , lane k; Supplementary Fig. 16 ), a phenomenon consistent with the previous report that Y723F mutation led to TOP1 SUMOylation at the K117 residue without CPT treatment [25] . 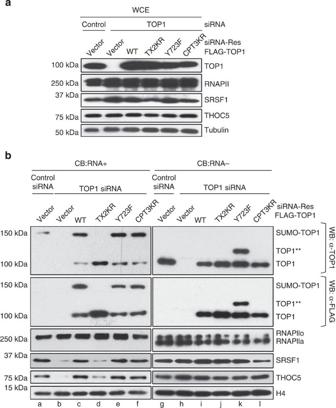Figure 6: TOP1 K391/K436 SUMOylation promotes the recruitment of RNA processing factors to actively transcribed regions. (a) The protein levels of TOP1, RNAPII, SRSF1 and THOC5 were analysed in WCEs prepared from control knockdown cells, TOP1 knockdown cells, and TOP1 knockdown cells complemented with vector alone, siRNA-resistant FLAG-TOP1 WT, TX2KR, Y723F or CPT3KR. Tubulin was used as the loading control. (b) Representative WB analysis of TOP1, FLAG-TOP1, RNAPII, SRSF1 and THOC5 in CB:RNA+ and CB:RNA− fractions prepared from cells ina. Histone H4 was used as the loading control. Protein band marked with `**' was a potential modified form of TOP1 specific to the Y723F mutant. Figure 6: TOP1 K391/K436 SUMOylation promotes the recruitment of RNA processing factors to actively transcribed regions. ( a ) The protein levels of TOP1, RNAPII, SRSF1 and THOC5 were analysed in WCEs prepared from control knockdown cells, TOP1 knockdown cells, and TOP1 knockdown cells complemented with vector alone, siRNA-resistant FLAG-TOP1 WT, TX2KR, Y723F or CPT3KR. Tubulin was used as the loading control. ( b ) Representative WB analysis of TOP1, FLAG-TOP1, RNAPII, SRSF1 and THOC5 in CB:RNA+ and CB:RNA− fractions prepared from cells in a . Histone H4 was used as the loading control. Protein band marked with `**' was a potential modified form of TOP1 specific to the Y723F mutant. Full size image R-loop accumulation in cells defective in TOP1 SUMOylation Previously, we showed that RECQ5 prevents transcription-associated DSBs ( Fig. 7a,b and Supplementary Fig. 17 ; ref. 15 ). Therefore, we asked whether the formation of R-loops contributes to the high level of DSBs in the RECQ5-depleted cells. Indeed, in RECQ5-depleted cells expressing RNase H ( Fig. 7a and Supplementary Fig. 17 ), which removes the RNA strand of the RNA:DNA hybrid without affecting the TOP1 SUMOylation status ( Fig. 8a , lanes a–d, CB:RNA+ fraction shown in the centre panel; Supplementary Fig. 17 ), the number of DNA breaks measured by native comet assays was significantly reduced ( Fig. 7b ). To further confirm the increase in R-loops in the RECQ5-depleted cells, we immunoprecipitated R-loops from genomic DNA isolated from either control or RECQ5 knockdown cells using an R-loop-specific S9.6 monoclonal antibody [4] , [29] , followed by real-time quantitative PCR. The R-loop Database ( http://rloop.bii.a-star.edu.sg ) predicted that exon 3 (EX3) of the β-actin ( ACTB ) gene locus has a high potential to form R-loops ( Fig. 7c ). Indeed, compared with the non-transcribed (NT) sequence located 5 kb upstream of the ACTB promoter, the EX3 sequence was highly enriched in R-loop immunoprecipitation (R–loop IP; Fig. 7d ). RNase H treatment of the isolated genomic DNA before R–loop IP effectively reduced the EX3 signal to a level similar to that observed with the NT sequence ( Fig. 7d ). Importantly, RECQ5-depleted cells showed an increase in R-loop formation within EX3 of the ACTB gene but not the NT region ( Fig. 7d , compare the black and grey bars). In addition to EX3, R-loops have also been observed immediately downstream of the ACTB poly-adenylation sequence, known as the 5′pause (5′P) site ( Fig. 7c ), and the formation of R-loops at the 5′P site is important for efficient transcription termination [4] . We found that R-loops also accumulated at the 5′P site in RECQ5-depleted cells, but to a lesser extent ( Fig. 7d ), and this may be due to the senataxin-dependent R-loop resolution that aids to alleviate R-loop accumulation at the 5′P site [4] . 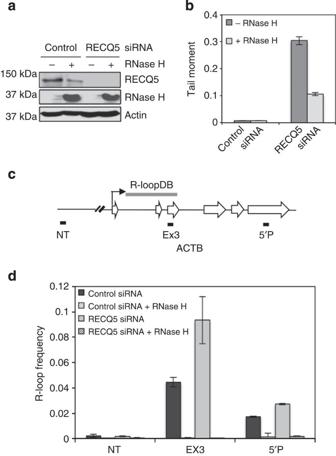Figure 7: R-loop-mediated DNA breaks in RECQ5-depleted cells. (a) The protein levels of RECQ5 and FLAG-RNase H were analysed in WCEs prepared from 293 T cells with or without transfection of pCMV-FLAG-RNase H plasmid. Actin was used as the loading control. (b) The average tail moment measured by the neutral comet assay using control and RECQ5 siRNA knockdown cells with or without RNase H expression froma. Each value is the mean tail moment±s.d. (n>200) per one representative experiment. (c) Diagram of theACTBgene structure. White arrows indicate the six exons and the black arrow indicates the transcription start site. The R-loop formation region predicted by R-loopDB is marked with a grey line. The NT region located 5 kb upstream of the ACTB promoter, EX3 and the 5′ pause site (5′P) were shown. (d) Representative analysis of the R-loop frequency at the NT, EX3 and 5′P sites in control and RECQ5 knockdown cells measured by R-loop IP using S9.6 antibody followed by quantitative PCR (qPCR) analysis. As a control, the isolated nucleic acids were treated with or without RNase H before R-loop IP. Each value represents the average value±standard deviation calculated from triplicate qPCRs per one representative experiment. Figure 7: R-loop-mediated DNA breaks in RECQ5-depleted cells. ( a ) The protein levels of RECQ5 and FLAG-RNase H were analysed in WCEs prepared from 293 T cells with or without transfection of pCMV-FLAG-RNase H plasmid. Actin was used as the loading control. ( b ) The average tail moment measured by the neutral comet assay using control and RECQ5 siRNA knockdown cells with or without RNase H expression from a . Each value is the mean tail moment±s.d. ( n >200) per one representative experiment. ( c ) Diagram of the ACTB gene structure. White arrows indicate the six exons and the black arrow indicates the transcription start site. The R-loop formation region predicted by R-loopDB is marked with a grey line. The NT region located 5 kb upstream of the ACTB promoter, EX3 and the 5′ pause site (5′P) were shown. ( d ) Representative analysis of the R-loop frequency at the NT, EX3 and 5′P sites in control and RECQ5 knockdown cells measured by R-loop IP using S9.6 antibody followed by quantitative PCR (qPCR) analysis. As a control, the isolated nucleic acids were treated with or without RNase H before R-loop IP. Each value represents the average value±standard deviation calculated from triplicate qPCRs per one representative experiment. 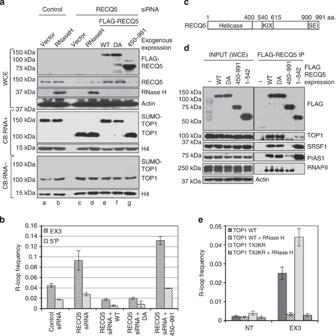Figure 8: The RECQ5 helicase domain is important for TOP1 SUMOylation and R-loop suppression. (a) (Top four panels) The protein levels of RECQ5, FLAG-RECQ5 and RNase H were analysed in WCEs prepared from control knockdown cells, RECQ5 knockdown cells and RECQ5 knockdown cells transfected with vector alone, FLAG-RNase H, siRNA-resistant FLAG-RECQ5 WT, ATPase-defective D157A (DA) mutant or the helicase domain-deleted 450–991 fragment. A rabbit α-RECQ5 antibody, which recognizes the helicase domain of RECQ5, cannot react with the RECQ5450–991fragment. Actin was used as the loading control. (Bottom four panels) WB analysis of TOP1 in the CB:RNA+ and CB:RNA− fractions prepared from the corresponding cells. Histone H4 was used as the loading control. (b) Representative analysis of the R-loop frequency at EX3 and 5′P sites in control, RECQ5 knockdown cells and RECQ5 knockdown cells complemented with RECQ5 WT, DA mutant or the 450–991 fragment measured by R-loop IP using isolated genomic DNA. Each value represents the average value±s.d. calculated from triplicate qPCR per one representative experiment. (c) Diagram of human RECQ5, its helicase domain and the RNAPII interaction domains (KIX and SRI). (d) Representative WB analysis of FLAG-RECQ5, TOP1, SRSF1, PIAS1 and RNAPII in WCE and in the immunopurified FLAG-RECQ5 WT, DA, 450–991 a.a. and 1–542 a.a. protein complexes. (e) Representative analysis of the R-loop frequency at NT and EX3 in TOP1 knockdown cells complemented with either siRNA-resistant FLAG-TOP1 WT or the TX2KR mutant with or without RNase H treatment before R-loop IP. Each value represents the average value±s.d. calculated from triplicate qPCRs per one representative experiment. Full size image Figure 8: The RECQ5 helicase domain is important for TOP1 SUMOylation and R-loop suppression. ( a ) (Top four panels) The protein levels of RECQ5, FLAG-RECQ5 and RNase H were analysed in WCEs prepared from control knockdown cells, RECQ5 knockdown cells and RECQ5 knockdown cells transfected with vector alone, FLAG-RNase H, siRNA-resistant FLAG-RECQ5 WT, ATPase-defective D157A (DA) mutant or the helicase domain-deleted 450–991 fragment. A rabbit α-RECQ5 antibody, which recognizes the helicase domain of RECQ5, cannot react with the RECQ5 450–991 fragment. Actin was used as the loading control. (Bottom four panels) WB analysis of TOP1 in the CB:RNA+ and CB:RNA− fractions prepared from the corresponding cells. Histone H4 was used as the loading control. ( b ) Representative analysis of the R-loop frequency at EX3 and 5′P sites in control, RECQ5 knockdown cells and RECQ5 knockdown cells complemented with RECQ5 WT, DA mutant or the 450–991 fragment measured by R-loop IP using isolated genomic DNA. Each value represents the average value±s.d. calculated from triplicate qPCR per one representative experiment. ( c ) Diagram of human RECQ5, its helicase domain and the RNAPII interaction domains (KIX and SRI). ( d ) Representative WB analysis of FLAG-RECQ5, TOP1, SRSF1, PIAS1 and RNAPII in WCE and in the immunopurified FLAG-RECQ5 WT, DA, 450–991 a.a. and 1–542 a.a. protein complexes. ( e ) Representative analysis of the R-loop frequency at NT and EX3 in TOP1 knockdown cells complemented with either siRNA-resistant FLAG-TOP1 WT or the TX2KR mutant with or without RNase H treatment before R-loop IP. Each value represents the average value±s.d. calculated from triplicate qPCRs per one representative experiment. Full size image Next we examined the cause of R-loop accumulation in the RECQ5 knockdown cells. We found that complementation with either the siRNA-resistant FLAG-RECQ5 WT or the ATPase-defective D157A (DA) mutant ( Fig. 8a , top panel, lanes e and f; Supplementary Fig. 17 ) successfully suppressed R-loop accumulation at the ACTB gene locus in the RECQ5 knockdown cells ( Fig. 8b ). This result is consistent with the previous report that RECQ5 is likely not directly involved in unwinding R-loops [20] . However, the helicase domain, but not the helicase activity, is still required for R-loop suppression, as demonstrated by the expression of the RECQ5 450–991 fragment, which lacks the helicase domain ( Fig. 8c ), in the RECQ5 knockdown cells ( Fig. 8a , top panel, lane g; Supplementary Fig. 17 and Fig. 8b ). Interestingly, although the RECQ5 knockdown cells complemented with the DA mutant showed normal TOP1 SUMOylation in the CB:RNA+ fraction, the expression of the RECQ5 450–991 fragment failed to rescue this defect ( Fig. 8a , centre panel; Supplementary Fig. 17 ). The defect in TOP1 SUMOylation is likely explained by the fact that the helicase domain located at the N terminus of RECQ5 is responsible for the interactions with the SRSF1-PIAS1 E3 ligase complex and TOP1 ( Fig. 8d and Supplementary Fig. 18 ). Since TOP1 SUMOylation promotes the efficient recruitment of RNA processing factors to the actively transcribed loci ( Fig. 6b ), it is possible that a failure to SUMOylate TOP1 during transcription contributed to R-loop accumulation in the RECQ5-deficient cells. In support of this conclusion, we found that the level of R-loops within EX3 of the ACTB gene, but not the NT region, was indeed elevated in the SUMOylation-defective TOP1 TX2KR mutant cells compared with the WT cells ( Fig. 8e ). Therefore, our results show that the helicase domain, but not the helicase activity, of RECQ5 is important for TOP1 SUMOylation, which facilitates the recruitment of RNA processing factors to the actively transcribed regions and minimizes R-loop formation. In human cells, we demonstrated that the TOP1 molecules are SUMOylated at K391 and K436 residues in a transcription-dependent but DNA damage-independent manner ( Figs 1 and 2 ). We further showed that the K391/K436 SUMOylation of TOP1 not only depends on the PIAS1 E3 ligase and its cofactor SRSF1 but also on the RECQ5 DNA helicase, and one mechanism by which RECQ5 induces the SUMOylation of TOP1 is to promote protein–protein interaction between TOP1 and PIAS1-SRSF1 ( Fig. 3 ). TOP1 is an essential enzyme in mammals [30] , and one of its primary functions during cell growth is to maintain DNA topology by relaxing supercoiled DNA [6] . TOP1 can localize to actively transcribed regions and associate with the RNAPIIo elongation complex in vertebrates [31] , [32] . Our analysis provides insight into the biological function of the TOP1 K391/K436 SUMO modifications during transcription. The exclusive localization of this SUMOylated form of TOP1 in the chromatin fraction that is enriched with proteins associated with highly transcribed DNA regions suggests that K391/K436 SUMOylation may have a role in the recruitment of TOP1 to the actively transcribed regions. However, the presence of unmodified TOP1 in the CB:RNA+ fraction in cells defective in K391/K436 SUMOylation ( Figs 3d and 6a ) argues that SUMOylation is not required for TOP1 localization to the highly transcribed regions. Most likely, those TOP1 molecules bound to the actively transcribed regions were recognized by RECQ5 and targeted to PIAS1-SRSF1-mediated SUMOylation. In cells defective in TOP1 SUMOylation, the TOP1 molecules at the actively transcribed regions remained unmodified. While K391/K436 SUMOylation is not required for TOP1 to associate with the highly transcribed regions, this transcription-induced modification is necessary for the direct physical interactions of TOP1 with the RNAPIIo elongation complex ( Figs 3 and 4 ) and the efficient recruitment of the RNA processing factors to the actively transcribed regions ( Fig. 6 ), a process that aids in suppressing genome instability caused by R-loop accumulation [1] , [2] , [10] . Indeed, cells defective in RECQ5-dependent TOP1 SUMOylation showed increased levels of R-loops and DSBs ( Figs 7 and 8 ). Negatively supercoiled DNA that forms during transcription also contributes to genomic instability by facilitating the formation of R-loops [33] . Unexpectedly, the TOP1 K391/K436 SUMO modifications that promote the recruitment of RNA processing factors to the actively transcribed regions significantly hinder the catalytic activity of TOP1 ( Fig. 5 ). The suppression of TOP1 activity is most likely due to the SUMO1 molecules conjugated to the TOP1 catalytic domain. Alternatively, because the SUMOylation promotes TOP1 protein–protein interactions, the suppression of the TOP1 catalytic activity may be achieved by the possible presence of the TOP1-interacting proteins co-purified with the WT, but not with the SUMOylation-defective TX2KR mutant. Our results indicate that TOP1 is dispensable for removing supercoiled DNA at these active transcription sites. It is possible that other topoisomerases, such as TOP3B, may function as the primary topoisomerase to relax negatively supercoiled DNA during transcription [34] . Because highly transcribed regions contain tandem arrays of RNAPIIo elongation complexes that move along the DNA template in the same direction, both positively and negatively supercoiled DNA can be generated between two juxtaposed RNAPIIo molecules. It is therefore also possible that these positive and negative supercoiled DNA could cancel each other out [35] . This could be a topoisomerase-independent method of regulating DNA supercoiling to avoid high levels of topoisomerase-induced genome instability during transcription. Our study may also provide important clues as to why RECQ5-deficient cells are hypersensitive to CPT but not other DNA-damaging agents [17] . In the RECQ5-depleted cells, the TOP1 molecules bound to the actively transcribed regions are not SUMOylated. These non-modified TOP1 molecules would have an active topoisomerase activity and could act on supercoiled DNA at highly transcribed regions of the chromosome, making these cells more susceptible to TOP1 poisons and the accumulation of TOP1–DNA covalent complexes. Unlike other members of the RECQ family of the DNA helicases, such as BLM, WRN and RECQ4, RECQ5 has not yet been definitively linked to any clinical diseases in the human population. Nevertheless, the importance of RECQ5 for preventing genome instability and reducing cancer risk has been clearly demonstrated in mice [12] . Interestingly, a recent study revealed that cells isolated from a sub-population of systemic sclerosis patients exhibit an unusual increase in SUMOylated TOP1 protein level and a decrease in TOP1 catalytic activity [36] . It would be of great interest to determine whether any of these abnormal SUMOylated TOP1 species can be linked to mutations in the RECQ5 gene, which would link RECQ5 to systemic sclerosis. In summary, our work provides evidence for a novel mechanism used by cells to balance the costs and benefits of relaxing supercoiled DNA by TOP1 for transcription. Plasmids TOP1 cDNA was PCR amplified from pYL1393-TOP1 (kindly provided by Dr Yung-Chi Cheng, Yale University) and cloned into pCMV-FLAG [13] between the EcoRI and BamHI sites. TOP1 mutants were generated by mutagenesis using a pCMV-FLAG-TOP1 WT plasmid as the template and the corresponding primers shown in Supplementary Table 1 . Full-length cDNAs encoding human RNase H1, PIAS1, SRSF1 and RPB3 were PCR amplified from a HeLa cDNA library and confirmed by DNA sequencing. RNase H1, PIAS1 and SRSF1 were cloned in pCMV-FLAG between the HindIII and EcoRI sites, whereas RPB3 was cloned between the HindII and BamHI sites. pCMV-FLAG-expressing siRNA-resistant RECQ5 WT was generated by mutagenesis using a pCMV-FLAG-RECQ5 WT plasmid as the template and the following primers: 5′-GCCAATGTCAGGTTTGTCGCACACTGGAACATCGCTAAATCCATGGCTGGGTACTACCAGG-3′. pCMV-FLAG-expressing siRNA-resistant RECQ5 1–542 and RECQ5 450–991 were constructed as described using siRNA-resistant pCMV-FLAG-RECQ5 WT plasmids [15] . The pCMV-FLAG-RECQ5 ATPase mutant, D157A (DA), was generated by mutagenesis using an siRNA-resistant pCMV-FLAG-RECQ5 WT plasmid as the template and the following primer: 5′-GAAGCTCATTGTGTTTCCCAATGGGCAGAAGCTCATTGTGTTTCCCAATGGG-3′. To generate GST-tagged SRSF1, full-length cDNAs was cloned into pGEX4T-1 between the BamHI and EcoRI sites, respectively. pET11-SUMO1 was kindly provided by Dr Yuan Chen (City of Hope). To generate the C-terminal 2xStrepII-tagged bacterial expression vector, pGEX-TwinStrep, the SalI-NotI fragment of pGEX4T-1 was replaced with a 130-bp SalI-NotI StrepTag II PCR fragment, 5′-GTCGACTCAGCGCTTGGAGCCACCCGCAGTTCGAGAAAGGTGGAGGTTCCGGAGGTGGATCGGGAGGTGGATCGTGGAGCCACCCGCAGTTCGAAAAATAAGCGGCCG-3′. To generate the GST-TOP1-StrepII expression plasmid, full-length cDNA was cloned into the above vector between EcoRI and BamHI. The GST-TOP1-StrepII K391R/K436R was generated by mutagenesis using the pGEX-TwinStrep-TOP1 plasmid as the template and the corresponding primers shown in Supplementary Table 1 . To generate GST-PIAS1-StrepII (for the pull-down experiments shown in Fig. 3f ), a full-length cDNA was cloned between the SalI and EcoRI sites, respectively. The chitin binding domain (CBD)-tagged RECQ5 was generated by cloning the full-length RECQ5 cDNA into pTXB1 between the Ndel and XhoI sites. Cell culture and transfection HEK293T cells were cultured in DMEM medium supplemented with 10% fetal bovine serum and streptomycin/penicillin (100 U ml −1 ). RECQ5 stealth siRNA 5′-UAGACUUGGCAAUAUUCCAAUGGGC-3′, TOP1 stealth siRNA 5′-GGGAAGGACUCCAUCAGAUACUAUA-3′, SRSF1 stealth siRNA 5′-UUAAGUUUACUGGCAUUGCTT-3′ and BLM stealth siRNA 5′-AUUCUAGGCAAUCAAAUGCCACCUU-3′ were purchased from Invitrogen. PIAS1 siRNA (sc-36219) was purchased from Santa Cruz. Plasmids and siRNAs were transfected using the Continuum Transfection Reagent (GEMINI) according to the manufacturer's protocol. When CPT or DRB were used, the concentrations were 5 and 25 μM, respectively. Antibodies Mouse α-GST (sc-138; 1:1,000), goat α-SRSF1 (sc-10254; 1:1,000), rabbit α-U2AF65 (sc-48804; 1:5,000), goat α-actin (sc-1616; 1:1,000), mouse α-tubulin (sc-8035; 1:3,000), goat α-BLM (sc-7790; 1:1,000), mouse α-SUMO1 (sc-5308; 1:1,000) and rabbit α-RNAPII (sc-899; 1:1,000) were purchased from Santa Cruz. Mouse α-RNAPII phospho-CTD (phospho S2; H5; ab24758; 1:5,000) and rabbit α-THOC5 (ab86070; 1:5,000) were purchased from Abcam. Rabbit α-Histone H4 (no. 2592; 1:1,000) and rabbit α-PIAS1 (no. 3550; 1:1,000) were purchased from Cell Signaling. Mouse α-NWSHPQFEK tag (StrepII tag; A01732; 1:3,000) was from GeneScript. Mouse α-p84 (GTX70220; 1:5,000) was from GeneTex and rabbit α-TOP1 (no. 3552-1; 1:5,000) was from Epitomics. Rabbit α-FLAG (F7425; 1:3,000) was purchased from Sigma-Aldrich. Mouse α-TOP1 (1:5,000) was kindly provided by Dr Yung-Chi Cheng (Yale School of Medicine). Mouse α-PCNA (1:5,000) was kindly provided by Dr Stephen West (Cancer Research UK). Rabbit α-RECQ5 (1:3,000) was generated as described [15] . Mouse α-DNA-RNA hybrid [S9.6] was kindly provided by Dr Stephen H. Leppla National Institutes of Health (NIH). Proteins GST, GST–PIAS1-StrepII (for the pull-down experiments shown in Fig. 3f ) and GST-SRSF1 were overexpressed in Escherichia coli for 12 h with 0.1 mM isopropyl β-D-1-thiogalactopyranoside (IPTG) at 16 °C. Cells were pelleted and resuspended in buffer A (1 × PBS, pH 7.4, 0.3 M NaCl, 0.5 mM EDTA, 1 mM dithiothreitol (DTT), 10% glycerol, 0.5% Triton X-100, protease inhibitor cocktail Complete (Roche)). Cells were lysed and debris was removed by centrifugation at 20,000 g for 30 min. Glutathione–agarose beads (Pierce) were incubated with the supernatant on a rocking platform for 2 h at 4 °C. After washing with 40 volumes of buffer A, bound proteins were eluted with 50 μl of elution buffer (50 mM glutathione, 50 mM Tris, pH 8.0, 0.3 M NaCl, 10% glycerol and 1 mM DTT) for three times. Fractions containing the protein were dialysed against buffer B (50 mM Tris, pH 8.0, 0.25 M NaCl, 10% glycerol, 1 mM DTT and 0.5 mM EDTA). GST-TOP1-StrepII was expressed in E. coli for 12 h after induction with 0.1 mM IPTG at 16 °C. Cells were pelleted and resuspended in buffer A. Cells were lysed and debris was removed by centrifugation at 20,000 × g for 30 min. Glutathione–agarose beads were incubated with the supernatant on a rocking platform for 2 h at 4 °C. After washing with 40 volumes of buffer A, bound proteins were eluted with 50 μl of elution buffer B for three times and incubated with Strep-Tactin resin (IBA) overnight at 4 °C. The beads were washed with five volumes of washing buffer (buffer B without glutathione). The proteins were eluted with washing buffer containing 2.5 mM desthiobiotin. The eluted proteins were collected and dialysed against buffer (50 mM Tris, pH 8.0, 0.25 M NaCl, 10% glycerol, 1 mM DTT and 0.5 mM EDTA). The expression of His-SUMO1 was induced for 4 h with 0.1 mM IPTG at 37 °C. Cells were pelleted and resuspended in buffer C (50 mM Tris, pH 8.0, 0.3 M NaCl, 0.5 mM EDTA, 1 mM DTT, 10% glycerol, 0.5% Triton X-100 and protease inhibitor cocktail Complete (Roche)). His-SUMO1 proteins were bound to Ni-NTA affinity resin (Qiagen), eluted by buffer C containing 200 mM imidazole and dialysed against buffer B (50 mM Tris, pH 8.0, 0.25 M NaCl, 10% glycerol, 1 mM DTT and 0.5 mM EDTA) before storage. RECQ5 was purified by Chitin Resin (New England Biolabs) and cleaved by DTT according to the manufacturer’s protocol (New England Biolabs) [18] . Cell fractionation and IP Cytoplasmic, nucleoplasmic and benzonase-treated soluble CB fractions were prepared as described [37] , except that N -ethylmalemide (40 mM) was included in the hypotonic lysis buffer to inhibit endogenous SUMO proteases and stabilize SUMO conjugates. The RNase A-sensitive soluble chromatin fraction (CB:RNA+) was prepared by digesting the chromatin pellet in RNase A buffer (50 mM Tris, pH 7.4, 10 mM EDTA, 150 mM NaCl, 10% glycerol, protease and phosphotease inhibitor) containing 250 μg ml −1 RNase A (Qiagen). After the supernatant (CB:RNA+ fraction) was collected, the pellet was further resuspended in nuclease incubation buffer (150 mM HEPES, pH 7.9, 1.5 mM MgCl 2 , 150 mM KCl, 10% glycerol, protease and phosphotease inhibitors) containing 0.15U μl −1 benzonase (Novagen). The sample was cleared by centrifugation at 20,000 g for 30 min, and the supernatant was collected as CB:RNA− fraction. For immunopurification of the FLAG-tagged protein complexes, extracts were incubated overnight with M2 agarose (Sigma) at 4 °C. After binding of the protein complexes, beads were washed extensively with and stored in FLAG-A-binding buffer (10 mM HEPES, pH 7.9, 1.5 mM MgCl 2 , 0.25 M NaCl, 10 mM KCl, 0.2% Triton X-100 and 10% glycerol) [37] . Topoisomerase assay The DNA relaxation activity assays using supercoiled plasmid pCMV-FLAG to monitor the activities of TOP1 were performed as described [38] . Briefly, in a 20-μl reaction mixture containing 50 mM Tris, pH 7.5, 100 mM KCl, 1 mM DTT, 10 mM EDTA and 5 μg ml −1 BSA, 0.2 μg of supercoiled plasmid DNA was relaxed by using the indicated amount of TOP1 at 37 °C for indicated amount of time. The reaction was stopped by addition of proteinase K for 30 min at 37 °C. The topological state of each DNA sample was analysed by electrophoresis in 1 × TAE buffer, pH 7.8, in a one-dimensional 1% agarose gel. Ethidium bromide (2 μg ml −1 ) was added to the corresponding reactions as negative controls. For the reactions shown in Fig. 5c , 0.5, 1 and 2 μl of the SUMO deconjugation reactions were used in the 20-μl DNA relaxation activity assays. In vitro SUMOylation and de-SUMOylation assays In vitro SUMOylation was carried out at 37 °C for 1 h using a SUMOylation kit and GST-PIAS1 proteins (without StrepII tag) purchased from Enzo Life Sciences, Inc. For each reaction, GST-TOP1 (250 ng) was incubated with the following proteins: SUMO E1 (25 ng), SUMO E2 (25 ng), SUMO1 (0.5 μg), PIAS1 (50 ng), SRSF1 (25 ng) or RECQ5 (50 ng). For SUMO deconjugation, SENP1 (BostonBiochem) was first pre-incubated in SENP buffer (50 mM Tris-HCl, pH. 7.5, 150 mM NaCl, 10% glycerol and 10 mM DTT) on ice for 30 min. The pre-incubated SENP1 was added into the SUMO deconjugation reaction (50 mM Tris-HCl, pH. 7.5, 150 mM NaCl, 10% glycerol and 5 mM DTT) at final concentration of 100 nM and incubated with the SUMOylated substrates at 30 °C for 8h [39] . In vitro protein interaction assays For FLAG-RPB3 pull down, after the SUMOylation reaction, an aliquot of the reaction was diluted with 10 volumes of FLAG binding buffer (10 mM HEPES, pH 7.9, 1.5 mM MgCl 2 , 0.20 M NaCl, 10 mM KCl, 0.2% Triton X-100 and 10% glycerol) incubated with FLAG-RNAPII purified from HEK293T cells using FLAG-RPB3 that remained bound to the M2 agarose beads for 4 h at 4 °C. After incubation and washing, the pull-down components were analysed by western immunoblotting. For the GST-TOP1 pull-down assay, the SUMOylation reaction was diluted with 10 volumes of Ni-NTA binding buffer (50 mM Tris, pH 8.0, 0.3 M NaCl, 10% glycerol, 0.1% Triton X-100 and 5 mM imidazole) and incubated with Ni-NTA beads overnight at 4 °C. The His-SUMO1-conjugated GST-TOP1 proteins were then eluted with Ni-NTA elution buffer (50 mM Tris, pH 8.0, 0.3 M NaCl, 10% glycerol, 0.1% Triton X-100 and 250 mM imidazole), dialysed against storage buffer (50 mM Tris, pH 8.0, 0.3 M NaCl, 10% glycerol, 1 mM EDTA and 1 mM DTT) and incubated with or without SENP1 at 30 °C for 8 h as described above [39] , before being immobilized on glutathione–agarose beads and incubated with FLAG–RNAPII complex purified from the CB:RNA+ fraction. After incubation and washing, the pull-down components were analysed by western immunoblotting. CBD pull down was performed as described with modification [40] . Briefly, CBD- and CBD-RECQ5-bound chitin beads were blocked with 1 mg ml −1 BSA in buffer D (40 mM Tris, pH 7.4, 10% glycerol, 0.1% Triton X-100, 1 mM EDTA, 150 mM NaCl and 1 mM DTT) for 30 min at 4 °C. GST, GST-TOP1, GST-SRSF1 or GST-PIAS1 were then added to the chitin beads and incubated for 2 h at 4 °C. The bound proteins were washed extensively with buffer D, boiled in SDS sample buffer, separated by SDS–PAGE, and analysed on western immunoblots. Neutral comet assays DNA breaks were analysed using neutral comet assays according to the manufacturer’s instructions (Trevigen, United Kingdom). Briefly, after RECQ5 siRNA and plasmid transfection, cells were harvested and resuspended in PBS at a density of 1 × 10 5 cells per ml. Samples were fixed in low-melting-point agarose and spread evenly onto a precoated slide. Samples were allowed to dry at 4 °C for 30 min, followed by cell lysis in prechilled lysis solution (Trevigen, United Kingdom) for 30 min at 4 °C in the dark. Slides were then washed in 1 × Tris-borate-EDTA buffer and electrophoresed at a constant voltage of 1 V cm −1 for 30 min. Slides were immersed in 70% ethanol for 5 min, air-dried, stained using SYBR green and air-dried for at least 24 h before viewing with a fluorescent microscope. The comet tail moment was recorded by randomly choosing 200 cells per slide using the Comet Assay IV software. R-loop IP R-loop IP was performed according to previous studies with modifications [4] , [5] , [34] . Briefly, total nucleic acids were extracted from 293 T cells by incubation with SDS/proteinase K buffer (50 mM Tris, pH 8.0, 10 mM EDTA, 0.5% SDS and 300 μg ml −1 proteinase K) at 37 °C overnight, followed by phenol/chloroform extraction and ethanol precipitation. Nucleic acids were fragmented using the restriction enzymes XbaI and SacI with or without RNase H at 37 °C overnight. After phenol/chloroform extraction and ethanol precipitation, 4 μg of nucleic acids per sample were immunoprecipitated with 2.5 μg of S9.6 antibody in binding buffer (10 mM NaPO 4 , pH 7.0, 140 mM NaCl and 0.05% Triton X-100) at 4 °C overnight. The binding complexes were then incubated with protein A agarose for 1 h at 4 °C and washed with binding buffer extensively. The bound nucleic acids were eluted with SDS/proteinase K buffer at 50 °C for 1 h, and purified by phenol/chloroform extraction and ethanol precipitation. Immunoprecipitated nucleic acids were quantified by quantitative PCR using the SYBR Green (Power) PCR Master Mix (Life Technologies) and the ABI 7500 Fast Real-Time PCR System. The primers used for upstream NT region of ACTB were 5′-CCCATCTGAAACATGGGGCT-3′ and 5′-GGCCAGGGAAAGTGAGAGAC-3′. The ACTB EX3 primers were 5′-GCTCAGGGCTTCTTGTCCTT-3′ and 5′-TCGATGGGGTACTTCAGGGT-3′. The ACTB 5′P primers were 5′-TTACCCAGAGTGCAGGTGTG-3′ and 5′-CCCCAATAAGCAGGAACAGA-3′. How to cite this article: Li, M. et al. RECQ5-dependent SUMOylation of DNA topoisomerase I prevents transcription-associated genome instability. Nat. Commun. 6:6720 doi: 10.1038/ncomms7720 (2015).